A novel Nrf2-miR-29-desmocollin-2 axis regulates desmosome function in keratinocytes The Nrf2 transcription factor controls the expression of genes involved in the antioxidant defense system. Here, we identified Nrf2 as a novel regulator of desmosomes in the epidermis through the regulation of microRNAs. On Nrf2 activation, expression of miR-29a and miR-29b increases in cultured human keratinocytes and in mouse epidermis. Chromatin immunoprecipitation identified the Mir29ab1 and Mir29b2c genes as direct Nrf2 targets in keratinocytes. While binding of Nrf2 to the Mir29ab1 gene activates expression of miR-29a and -b, the Mir29b2c gene is silenced by DNA methylation. We identified desmocollin-2 (Dsc2) as a major target of Nrf2-induced miR-29s. This is functionally important, since Nrf2 activation in keratinocytes of transgenic mice causes structural alterations of epidermal desmosomes. Furthermore, the overexpression of miR-29a/b or knockdown of Dsc2 impairs the formation of hyper-adhesive desmosomes in keratinocytes, whereas Dsc2 overexpression has the opposite effect. These results demonstrate that a novel Nrf2-miR-29-Dsc2 axis controls desmosome function and cutaneous homeostasis. Nuclear factor erythroid 2-related factor 2 (Nrf2), a member of the cap ‘n’ collar family of transcription factors, is well known for its key role in the cellular antioxidant defense [1] , [2] . This activity is very important in the skin, where loss of Nrf2 or its functional inhibition prolonged the inflammatory response after wounding [3] and enhanced the susceptibility to chemically induced carcinogenesis [4] , [5] . On the other hand, Nrf2 is activated in a variety of human cancers [6] , including cutaneous squamous cell carcinomas [7] , and activation of Nrf2 correlates with increased tumour aggressiveness [4] , [8] . Furthermore, we recently showed that pharmacological or genetic activation of Nrf2 in keratinocytes of mouse skin severely affects the cornified enveloping, resulting in the development of an ichthyosis-like skin disease that is characterized by acanthosis, hyperkeratosis and impaired barrier function [9] . It is therefore essential to examine the consequences of Nrf2 activation in physiological and pathological contexts and to identify the responsible Nrf2 target genes. Nrf2 is expressed in most cell types and particularly high levels are seen in epithelial cells that are exposed to the environment, such as keratinocytes [1] , [3] . Its activity is strongly enhanced in response to electrophilic and oxidative stress, which results in stabilization and nuclear accumulation of Nrf2 (ref. 10 ). Induction of gene expression occurs through binding of Nrf2 in combination with a small Maf protein or other binding partners to so-called antioxidant response elements (ARE) in the promoters or enhancers of target genes [2] , [11] , [12] . The biological effects of Nrf2 may depend on the level of Nrf2 activation, its binding partners, and, as a result, on different sets of target genes activated by Nrf2 at the level of transcription. Interestingly, the transcriptional activity of Nrf2 is not restricted to genes involved in the antioxidant defense. Rather, it also controls expression of genes with other functions, such as regulation of cell proliferation and survival [13] . Chromatin immunoprecipitation followed by sequencing (ChIP-Seq) revealed that Nrf2 binds to promoters of genes encoding microRNAs (miRNAs, miRs) [13] , [14] , [15] , although the functional consequences remain largely unknown. Binding of Nrf2 to AREs usually results in the activation of gene expression, but Nrf2 also represses a few genes through as yet poorly characterized mechanisms [16] , [17] , [18] , [19] . We therefore speculated that some of these genes are targets of Nrf2-activated miRNAs. Together with protein-coding genes, miRNAs are involved in the integration of multiple signalling pathways. They are small, single-stranded, non-coding RNAs that bind to the 3′-untranslated region (3′UTR) of target mRNAs [20] . Conditional deletion of genes encoding Dicer and DiGeorge syndrome critical region gene 8 (Dgcr8), key proteins involved in miRNA biogenesis, revealed important roles of miRNAs in mammalian skin development and function [21] , [22] . Furthermore, miRNAs are regulators of keratinocyte proliferation and differentiation in normal and wounded skin, as well as in autoimmune and chronic skin diseases [23] , [24] , [25] . Therefore, we decided to study the role of Nrf2 in the control of miRNA expression in the skin. Here, we show that Nrf2 activates expression of miR-29a and miR-29b in keratinocytes. This occurs through direct binding and transcription activation of the Mir29ab1 gene, whereas the Mir29b2c gene is silenced in keratinocytes by DNA methylation. The upregulation of these miRs is functionally important, since miR-29a and -b target desmocollin-2, a major desmosomal component. The reduction in desmocollin-2 (Dsc2) impairs desmosome hyper-adhesiveness in keratinocytes. These results identify a novel miR-29-Dsc2 axis in keratinocytes, which controls desmosome function in the epidermis. Nrf2 regulates expression of miR-29s in mouse skin To identify Nrf2-regulated miRs in keratinocytes, we made use of transgenic mice expressing a constitutively active mutant of Nrf2 (caNrf2) under the control of a cytomegalovirus enhancer (CMV) and a β-actin promoter. To avoid constitutive expression of the transgene, the caNrf2 cDNA is preceded by a floxed STOP cassette. On mating these mice with transgenic mice expressing Cre recombinase under control of a keratin 5 (K5) promoter, the STOP cassette is deleted in keratinocytes, resulting in expression of caNrf2 in all layers of the epidermis and in the hair follicles. The double mutant mice (designated K5Cre-CMVcaNrf2 mice) develop progressive epidermal thickening and hyperkeratosis as well as enlarged sebaceous glands [9] , [26] . However, only very minor phenotypic abnormalities are present in neonatal mice [9] . We therefore used the back skin of K5Cre-CMVcaNrf2 mice and littermate controls at P2.5 to identify direct miR targets of Nrf2 using microarray analysis ( Supplementary Data 1 ). Transgenic mice expressing a dominant-negative mutant of Nrf2 (dnNrf2) in keratinocytes (K14-dnNrf2 mice) [5] were used as additional control. Since dnNrf2 lacks the transactivation domain, this allowed us to determine whether miRNA expression is dependent on the transcriptional activity of Nrf2. We found a significant increase in the levels of miR-494, miR-29a, miR-29b, miR-29c and miR-672 in the skin of K5cre-CMVcaNrf2 compared with control littermates ( Fig. 1a ). TaqMan-based quantitative PCR (qPCR) analysis confirmed the upregulation of miR-29a, miR-29b and miR-29c ( Fig. 1b ). These miRs were not upregulated in K14-dnNrf2 transgenic mice at P2.5, suggesting that Nrf2 regulates miR-29s at the level of transcription ( Fig. 1c ). The increase in the expression of miR-29s was even more pronounced at P32, when the phenotype of the K5Cre-CMVcaNrf2 mice had developed. At this time point, we observed a downregulation in K14-dnNrf2 mice ( Fig. 1d ), indicating that endogenous Nrf2 also controls miR-29s expression. The Nrf2-induced upregulation of miR-29s is a cell autonomous effect, since it was also observed in cultured primary keratinocytes from K5Cre-CMVcaNrf2 mice ( Fig. 1e ). 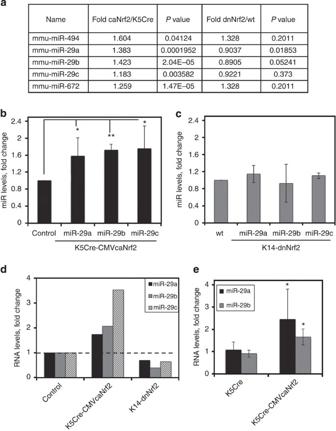Figure 1: Nrf2 regulates the expression of the miR-29 family in mouse skin. (a) List of miRNAs significantly upregulated in the skin of K5Cre-CMVcaNrf2 mice as detected by miRNA microarray analysis using RNAs from K5Cre (control), K5Cre-CMVcaNrf2, wild-type and K14-dnNrf2 mice (N=3 per genotype). (b) Levels of mature miR-29s measured by TaqMan assays in skin of control and K5Cre-CMVcaNrf2 mice at P2.5 (N=8) (b) and of K14-dnNrf2 and wild-type mice at P2.5 (N=5) (c). (d) Levels of miR-29s were measured in the skin of K5Cre, and of K5Cre-CMVcaNrf2 and K14-dnNrf2 mice at P32. The experiment was performed with two independent pools of RNAs from three littermates per genotype. A representative experiment is shown. Note the increase in miR-29s in K5Cre-CMVcaNrf2 mice and the reduction in K14-dnNrf2 mice at P32. (e) Levels of mature miR-29s measured by TaqMan assays in primary keratinocytes isolated from K5Cre and K5Cre-CMVcaNrf2 mice at P4.5 (N=5). Error bars represent s.d.,t-testPvalue *<0.05; **<0.01. Figure 1: Nrf2 regulates the expression of the miR-29 family in mouse skin. ( a ) List of miRNAs significantly upregulated in the skin of K5Cre-CMVcaNrf2 mice as detected by miRNA microarray analysis using RNAs from K5Cre (control), K5Cre-CMVcaNrf2, wild-type and K14-dnNrf2 mice ( N =3 per genotype). ( b ) Levels of mature miR-29s measured by TaqMan assays in skin of control and K5Cre-CMVcaNrf2 mice at P2.5 ( N =8) ( b ) and of K14-dnNrf2 and wild-type mice at P2.5 ( N =5) ( c ). ( d ) Levels of miR-29s were measured in the skin of K5Cre, and of K5Cre-CMVcaNrf2 and K14-dnNrf2 mice at P32. The experiment was performed with two independent pools of RNAs from three littermates per genotype. A representative experiment is shown. Note the increase in miR-29s in K5Cre-CMVcaNrf2 mice and the reduction in K14-dnNrf2 mice at P32. ( e ) Levels of mature miR-29s measured by TaqMan assays in primary keratinocytes isolated from K5Cre and K5Cre-CMVcaNrf2 mice at P4.5 ( N =5). Error bars represent s.d., t -test P value *<0.05; **<0.01. Full size image The genes encoding miR-29s are direct Nrf2 targets MiR-29s are encoded by two gene clusters ( Mir29ab1 and Mir29b2c ) in mice and humans ( Figs 2a and 3a ). Both clusters can give rise to mature miR-29b, whereas sequences coding for miR-29a and miR-29c are not duplicated. Using bioinformatics, we identified DNA-binding sites for Nrf2 (AREs) within ~25 kb upstream of the sequences encoding miR-29s in mice ( Figs 2a and 3a and Supplementary Fig. 1A ). Earlier, RACE analysis had identified transcription start sites (TSS) for the human MIR29AB1 and MIR29B2C clusters, and based on conservation analysis and ENCODE data, we predicted the TSS for the mouse Mir29ab1 and Mir29b2c genes approximately in the same positions upstream of the sequences encoding miR-29s (ref. 27 ). According to the current annotation [27] , the identified AREs are located within genes encoding the long non-coding RNAs (lncRNAs) MIR-29A-001 and C1ORF132 in humans ( Figs 2a and 3a ). 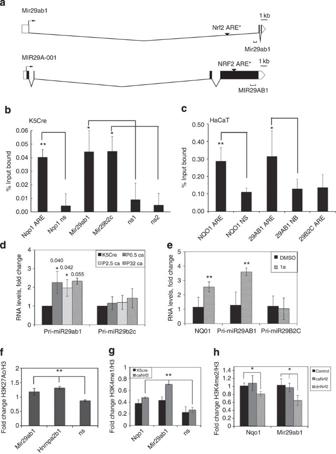Figure 2: Nrf2 binds and activates enhancer elements of mouse and humanmiR-29a/b1genes. (a) Diagram showing the locations of Nrf2-bound AREs in the 5′ regions of the mouseMir29ab1(top) and humanMIR29AB1(bottom) genes. Note that the humanMIR29AB1cluster is located within the annotated lncRNA MIR-29A-001, whereas the location of the TSS of mouseMir29ab1is based on conservation analysis27. The TSS of the human gene and the predicted TSS of the murine gene are indicated with bent arrows. (b,c) Nrf2 binds to the AREs of theMir29ab1andMIR29AB1genes in the epidermis of K5Cre mice (b) and in human keratinocytes treated with compound1a(c). Primers used for ChIP experiments hybridized to the AREs marked with the asterisks ina. Binding of Nrf2 to the ARE ofNqo1served as a positive control. Primers spanning a ns region located 2 kb away from the ARE of each gene were used as negative control. The average of at least three independent ChIP experiments is shown as percentage of input bound. (d) Levels of primary transcripts of theMir29ab1and theMir29b2cgenes (Pri-miR29ab1 and Pri-miR29bc2) were measured in the skin of control and K5Cre-CMVcaNrf2 mice at P0.5, P2.5 and P32 by qPCR (N=5 per genotype and time point). (e) Expression ofNQO1,Pri-MIRAB1andPri-MIRB2Cwas analysed by qRT-PCR in HaCaT cells treated with compound1a.N=3. (f–h) ChIPs using antibodies against total histone H3 and the modified histones H3K27Ac (f) or H3K4me1/2 (g,h) using epidermal lysates from K5Cre (f) K5Cre-CMVcaNrf2 (f–h) and K14-dnNrf2 mice (h). For H3K27Ac analysis, the promoter of theHnrnpa2gene served as a positive control. Non-specific control regions (ns) were used as negative controls. The average of the values from at least three independent ChIP experiments is calculated as percentage of input bound and as a fold of H3K27Ac, H3K4me1 or H3K4me2 over total histone H3 occupancy. Error bars represent s.d.,t-testPvalue *<0.05; **<0.01. RT–PCR, reverse transcriptase-PCR. Figure 2: Nrf2 binds and activates enhancer elements of mouse and human miR-29a/b1 genes. ( a ) Diagram showing the locations of Nrf2-bound AREs in the 5′ regions of the mouse Mir29ab1 (top) and human MIR29AB1 (bottom) genes. Note that the human MIR29AB1 cluster is located within the annotated lncRNA MIR-29A-001, whereas the location of the TSS of mouse Mir29ab1 is based on conservation analysis [27] . The TSS of the human gene and the predicted TSS of the murine gene are indicated with bent arrows. ( b , c ) Nrf2 binds to the AREs of the Mir29ab1 and MIR29AB1 genes in the epidermis of K5Cre mice ( b ) and in human keratinocytes treated with compound 1a ( c ). Primers used for ChIP experiments hybridized to the AREs marked with the asterisks in a . Binding of Nrf2 to the ARE of Nqo1 served as a positive control. Primers spanning a ns region located 2 kb away from the ARE of each gene were used as negative control. The average of at least three independent ChIP experiments is shown as percentage of input bound. ( d ) Levels of primary transcripts of the Mir29ab1 and the Mir29b2c genes (Pri-miR29ab1 and Pri-miR29bc2) were measured in the skin of control and K5Cre-CMVcaNrf2 mice at P0.5, P2.5 and P32 by qPCR ( N =5 per genotype and time point). ( e ) Expression of NQO1 , Pri-MIRAB1 and Pri-MIRB2C was analysed by qRT-PCR in HaCaT cells treated with compound 1a . N =3. ( f – h ) ChIPs using antibodies against total histone H3 and the modified histones H3K27Ac ( f ) or H3K4me1/2 ( g , h ) using epidermal lysates from K5Cre ( f ) K5Cre-CMVcaNrf2 ( f – h ) and K14-dnNrf2 mice ( h ). For H3K27Ac analysis, the promoter of the Hnrnpa2 gene served as a positive control. Non-specific control regions (ns) were used as negative controls. The average of the values from at least three independent ChIP experiments is calculated as percentage of input bound and as a fold of H3K27Ac, H3K4me1 or H3K4me2 over total histone H3 occupancy. Error bars represent s.d., t -test P value *<0.05; **<0.01. RT–PCR, reverse transcriptase-PCR. 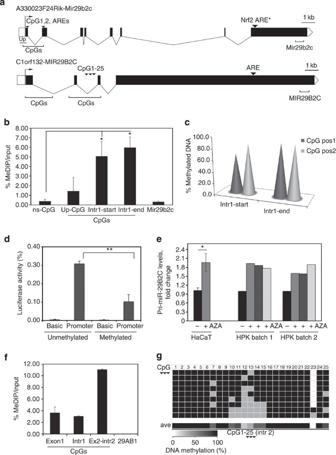Figure 3: TheMir29b2cgene is silenced by methylation in keratinocytes. (a) Location of CpGs at the promoter region of the mouseA330023F24Rikgene harbouring theMir29b2ccluster and of the humanC1ORF132gene containing theMIR29B2Ccluster. Positions of AREs within the last exon of both genes (bound by Nrf2 in mouse keratinocytes, but not in human keratinocytes) are indicated; single CpGs chosen for validation by bisulfite conversion are indicated (CpG1,2 forA330023F24Rikand CpG1-25 forC1ORF132). The murine CpG region also contains two AREs not bound by Nrf2 (AREs). (b) MeDIP analysis of DNA from mouse epidermis showing enrichment of methylated DNA in intron 1 of theA330023F24Rikgene compared with the region >2 kb away from the CpGs (ns-CpG). Levels of DNA methylation of control genes used for MeDIP are shown inSupplementary Fig. 2C. (c) Bisulfite conversion and pyrosequencing analysis of the DNA from mouse epidermis shows highly methylated single CpGs at positions 1 and 2 indicated ina. (d) The promoter region (2.5 kb) of theA330023F24RiklincRNA was cloned into a CpG-free pCpGL reporter vector, subjected toin vitromethylation, and luciferase activity was measured in cells transfected with the plasmid harbouring the methylated or non-methylated promoter. The basic CpG-free vector without promoter was used as negative control, the pCpGL vector with a CMV promoter served as positive control.N=4. (e) HaCaT cells and primary human keratinocytes (HPKs) were treated with DMSO (−AZA) or 5-aza-2′-deoxyuridine (+AZA), and levels of primary miR29B2C transcripts were measured by qRT-PCR. HaCaT cells were analysed in triplicates; two independent batches of human primary keratinocytes were analysed. (f) MeDIP analysis of the DNA isolated from primary human keratinocytes shows significant enrichment of methylated DNA in exon 1–intron 2 of theC1ORF132gene. DNA methylation of control genes used for MeDIP are shown inSupplementary Fig. 2H. The NRF2-bound ARE ofMIR29AB1was used as negative control. (g) Bisulfite sequencing of the DNA from HPKs shows highly methylated CpGs at positions 1–25 (also indicated inainside intron 2). Error bars represent s.d.,t-testPvalue *<0.05; **<0.01. RT–PCR, reverse transcriptase-PCR. Full size image Figure 3: The Mir29b2c gene is silenced by methylation in keratinocytes. ( a ) Location of CpGs at the promoter region of the mouse A330023F24Rik gene harbouring the Mir29b2c cluster and of the human C1ORF132 gene containing the MIR29B2C cluster. Positions of AREs within the last exon of both genes (bound by Nrf2 in mouse keratinocytes, but not in human keratinocytes) are indicated; single CpGs chosen for validation by bisulfite conversion are indicated (CpG1,2 for A330023F24Rik and CpG1-25 for C1ORF132 ). The murine CpG region also contains two AREs not bound by Nrf2 (AREs). ( b ) MeDIP analysis of DNA from mouse epidermis showing enrichment of methylated DNA in intron 1 of the A330023F24Rik gene compared with the region >2 kb away from the CpGs (ns-CpG). Levels of DNA methylation of control genes used for MeDIP are shown in Supplementary Fig. 2C . ( c ) Bisulfite conversion and pyrosequencing analysis of the DNA from mouse epidermis shows highly methylated single CpGs at positions 1 and 2 indicated in a . ( d ) The promoter region (2.5 kb) of the A330023F24Rik lincRNA was cloned into a CpG-free pCpGL reporter vector, subjected to in vitro methylation, and luciferase activity was measured in cells transfected with the plasmid harbouring the methylated or non-methylated promoter. The basic CpG-free vector without promoter was used as negative control, the pCpGL vector with a CMV promoter served as positive control. N =4. ( e ) HaCaT cells and primary human keratinocytes (HPKs) were treated with DMSO (−AZA) or 5-aza-2′-deoxyuridine (+AZA), and levels of primary miR29B2C transcripts were measured by qRT-PCR. HaCaT cells were analysed in triplicates; two independent batches of human primary keratinocytes were analysed. ( f ) MeDIP analysis of the DNA isolated from primary human keratinocytes shows significant enrichment of methylated DNA in exon 1–intron 2 of the C1ORF132 gene. DNA methylation of control genes used for MeDIP are shown in Supplementary Fig. 2H . The NRF2-bound ARE of MIR29AB1 was used as negative control. ( g ) Bisulfite sequencing of the DNA from HPKs shows highly methylated CpGs at positions 1–25 (also indicated in a inside intron 2). Error bars represent s.d., t -test P value *<0.05; **<0.01. RT–PCR, reverse transcriptase-PCR. Full size image ChIP analysis using an Nrf2-specific antibody [9] , [28] and epidermal lysates revealed that significantly more total Nrf2 (wild-type Nrf2, caNrf2 or dnNrf2) was bound to the AREs located −3.9 kb upstream of the sequences encoding miR-29a and -b ( Mir29ab1 gene) and −2.8 kb upstream of the sequences encoding miR-29b and -c ( Mir29b2c gene), compared with the non-specific (ns) control regions void of AREs ( Fig. 2b and Supplementary Fig. 1B–D ). The ARE located in the promoter region of the NAD(P)H dehydrogenase quinone 1 ( Nqo1 ) gene, a classical Nrf2 target gene, was used as a positive control. As expected, more total Nrf2 was bound to all tested AREs in K5Cre-CMVcaNrf2 mice ( Supplementary Fig. 1B,C ) and K14-dnNrf2 mice ( Supplementary Fig. 1D ) than in control mice ( Fig. 2b ), although the difference compared with the ns binding was similar in mice of all genotypes. The result obtained with epidermis from K5Cre-CMVcaNrf2 mice was reproduced with an independent antibody ( Supplementary Fig. 1B,C ). When we activated endogenous NRF2 in primary human keratinocytes with a non-toxic small molecule (compound 1a (ref. 29 )), we detected binding of NRF2 to the ARE located at −2.5 kb upstream of the MIR29AB1 gene, but not to the ARE of the MIR29B2C gene ( Fig. 2c ). Consistent with the data obtained for the mature miRs, levels of the Mir29ab1 primary transcript increased in the skin of K5Cre-CMVcaNrf2 mice at P0.5, P2.5 and P32 ( Fig. 2d ). The expression of pri-miR29AB1 also increased after the activation of NRF2 with compound 1a ( Fig. 2e ). However, expression of the primary transcript of the Mir29b2c gene was not induced by caNrf2 in vivo ( Fig. 2d ). This finding also demonstrates that the apparent upregulation of miR-29c in K5Cre-CMVcaNrf2 mice ( Fig. 1b ) resulted from detection of the highly homologous miR-29a by the Taqman assay (Life Technologies, personal communication). Similar to the situation in the mouse, compound 1a did not activate transcription of the human MIR29B2C gene ( Fig. 2e ). This can be explained by the lack of NRF2 binding at the MIR29B2C cluster. However, the failure of Nrf2 to activate expression of the mouse Mir29b2c gene required further investigation. To further characterize the mechanism of Nrf2-induced expression of Mir29ab1 , we analysed marks of active enhancers across the upstream sequences of the Mir29 clusters by ChIP analysis. Histone H3K27 acetylation (H3K27Ac) as well as H3K4 mono- and dimethylation (H3K4me1 and H3K4me2), epigenetic marks of active promoter and enhancer elements [30] , showed higher occupancy at the Mir29ab1 ARE compared with the ns site ( Fig. 2f,g and Supplementary Fig. 1E,F ). The occupancy of H3K27Ac at the ARE of the Mir29ab1 cluster was comparable to the occupancy at the active promoter/enhancer element of the gene encoding heterogeneous nuclear ribonucleoprotein A2/B1 ( Hnrnpa2b1 ) [31] , and H3K4me2 occupancy at the ARE of the Mir29ab1 cluster was comparable to the Nqo1 ARE, indicating a transcriptionally active state of chromatin at this site in control and K5Cre-CMVcaNrf2 mice ( Fig. 2h ). Importantly, dnNrf2 caused a significant reduction in H3K4me2 levels ( Fig. 2h ), suggesting that the transcriptional activity of Nrf2 is required to activate this site. The presence of the H3K4me2 mark at the Mir29b2c ARE was, however, much lower ( Supplementary Fig. 1E,F ), indicating a closed chromatin conformation. H3K4me2 levels were higher at the Mir29b2c ARE in K5Cre-CMVcaNrf2 mice compared with K5Cre control mice ( Supplementary Fig. 1E ), but this was obviously insufficient for transcriptional activation. Thus, Nrf2 activates expression of miR-29s through direct binding and transcriptional activation of the Mir29ab1 cluster, whereas binding of Nrf2 to the ARE of the Mir29b2c gene does not activate its expression in mouse keratinocytes. The Mir29b2c cluster is silenced by DNA methylation Previous studies identified a TSS of the human MIR29B2C cluster at −20 kb upstream of the stem-loop sequences of miR-29b2/c and demonstrated high genomic conservation of the regulatory elements in this region between mice and humans [27] , [32] . The Mir29b2c cluster resides inside the last exon of the lncRNA A330023F24Rik , and the human MIR29B2C cluster locates within the last exon of lncRNA C1ORF132 ( Fig. 3a ). 5′RACE [27] and analysis of ChIP-seq data available from the ENCODE project predicted promoters, which are located immediately at the 5′ end of the A330023F24Rik and C1ORF132 genes, and ~20 kb upstream of the highly conserved sequence encoding miR-29b2/c ( Fig. 3a and Supplementary Fig. 2A,B ). This promoter is characterized by a strong peak of H3K4me3 and polymerase II binding in several cell types and tissues ( Supplementary Fig. 2A,B ) and is therefore most likely responsible for the initiation of the transcription of the mouse Mir29b2c gene. We speculated that this −20 kb TSS is subject to epigenetic silencing in keratinocytes. Consistent with this hypothesis, we identified CpG-rich areas (islands) immediately downstream of the TSS of the A330023F24Rik and C1ORF132 genes ( Fig. 3a and Supplementary Fig. 2A,B ). Using methylated DNA immunoprecipitation (MeDIP) and bisulfite-treated DNA sequencing, we detected strong DNA methylation (78–91%) at this region in mouse epidermis in vivo ( Fig. 3b,c , Supplementary Fig. 2C,D ) and in cultured mouse keratinocytes (91–94%; Supplementary Fig. 2D ). Importantly, the unmethylated A330023F24Rik promoter was able to activate the expression of a reporter gene, which was abrogated when the CpGs were methylated in vitro ( Fig. 3d ). We also found that the Nrf2-bound ARE further downstream acts as a functional enhancer when cloned into a reporter plasmid with a minimal promoter, as demonstrated by the strong increase in luciferase activity on transfection with a caNrf2 expression vector ( Supplementary Fig. 2E ). However, the lack of Nrf2 binding to AREs present in the promoter region of A330023F24Rik ( Fig. 3a ) as well as low H3K4me2/3 levels confirmed an inactive state of the chromatin at the A330023F24Rik TSS ( Supplementary Fig. 2G,F ). These results suggest that Nrf2 activates the Mir29b2c cluster in a methylation-free context, but that DNA methylation prevents activation of the cluster. The DNA methylation-dependent silencing mechanism is conserved in the human C1ORF132 gene as demonstrated by the increase in pri-miR-29B2/C levels following demethylation of the DNA by treatment of human keratinocytes with 5-aza-2′-deoxyuridine ( Fig. 3e ). MeDIP and bisulfite conversion followed by sequencing of the CpG islands of the C1ORF132 gene revealed that >86% of the DNA was methylated in primary human keratinocytes ( Fig. 3f,g and Supplementary Fig. 2I ). A novel role of Nrf2 in the control of desmosome function To identify the targets of Nrf2-regulated miR-29a and -b in keratinocytes, which mediate Nrf2 function, we first performed a bioinformatics analysis to identify predicted miR-29 targets that are expressed in the skin. At least 4,707 mRNAs were identified that fulfill this criterion ( Fig. 4a and Supplementary Data 2 ). Pathway analysis revealed that many of them encode proteins that are involved in cell–cell and cell–matrix adhesion ( Fig. 4b and Supplementary Fig. 3A ). A comparison of the predicted targets with the mRNAs that are downregulated in the skin of K5Cre-CMVcaNrf2 mice [9] identified various desmosomal components, including Dsc2 and desmoglein 2 ( Supplementary Fig. 3B ). Consistent with this finding, ultrastructural analysis of the epidermis of K5Cre-CMVcaNrf2 mice revealed obvious desmosomal abnormalities. There was an increased distance between desmosomal plaques of two neighbouring keratinocytes that was due to enlargement of the desmosomal core ( Fig. 4c ). Furthermore, most of the desmosomes in control mice had a midline that reflects ‘hyper-adhesiveness’ [33] , whereas a midline could not be detected in most of the desmosomes of K5Cre-CMVcaNrf2 mice ( Fig. 4c ). 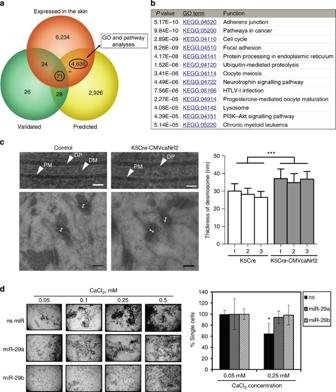Figure 4: Nrf2 and miR-29s regulate desmosomes. (a) Functional annotation and pathway analyses of 4,707 genes from the Venn diagram representing mRNAs highly expressed in the skin (Expressed in the skin), mRNAs predicted to be targets of miR-29s (Predicted), and mRNAs shown to be targets of miR-29s based on the literature (Validated;Supplementary Data 2). (b) KEGG pathway analysis based on 4,707 genes expressed in the skin and potentially regulated by miR-29s, as indicated ina. (c) Ultrastructural analysis of sections from K5Cre and K5Cre-CMVcaNrf2 mouse skin at P32. Representative micrographs of a single desmosome (upper panel, scale bar 30 nm) and of a field with several desmosomes in the skin of control and K5Cre-CMVcaNrf2 mice (lower panel; scale bar, 150 nm). DM, dense midline, PM, plasma membrane; DP, dense plaque. Note the absence of a DM, the thicker DP, and the wider distance between opposing PMs in K5Cre-CMVcaNrf2 mice. Right panel: the thickness of desmosomes was calculated by comparing the distance between two opposing PMs (N=3 mice per genotype; 25–38 measurements per mouse). (d) Impaired formation of desmosomes by HaCaT cells transfected with miR-29. Seventy-two hours post transfection, cells were separated into a single-cell suspension in ethylene glycol tetraacetic acid-containing medium and then exposed to increasing concentrations of CaCl2to induce formation of desmosomes. Living single cells were stained with Trypan blue and counted in triplicate wells. No significant change in the number of single cells reflects impaired formation of desmosomes. Scale bars, 1 mm. Error bars represent s.d.,t-testPvalue *<0.05; two-way analysis of variance ***<0.001). Figure 4: Nrf2 and miR-29s regulate desmosomes. ( a ) Functional annotation and pathway analyses of 4,707 genes from the Venn diagram representing mRNAs highly expressed in the skin (Expressed in the skin), mRNAs predicted to be targets of miR-29s (Predicted), and mRNAs shown to be targets of miR-29s based on the literature (Validated; Supplementary Data 2 ). ( b ) KEGG pathway analysis based on 4,707 genes expressed in the skin and potentially regulated by miR-29s, as indicated in a . ( c ) Ultrastructural analysis of sections from K5Cre and K5Cre-CMVcaNrf2 mouse skin at P32. Representative micrographs of a single desmosome (upper panel, scale bar 30 nm) and of a field with several desmosomes in the skin of control and K5Cre-CMVcaNrf2 mice (lower panel; scale bar, 150 nm). DM, dense midline, PM, plasma membrane; DP, dense plaque. Note the absence of a DM, the thicker DP, and the wider distance between opposing PMs in K5Cre-CMVcaNrf2 mice. Right panel: the thickness of desmosomes was calculated by comparing the distance between two opposing PMs ( N =3 mice per genotype; 25–38 measurements per mouse). ( d ) Impaired formation of desmosomes by HaCaT cells transfected with miR-29. Seventy-two hours post transfection, cells were separated into a single-cell suspension in ethylene glycol tetraacetic acid-containing medium and then exposed to increasing concentrations of CaCl 2 to induce formation of desmosomes. Living single cells were stained with Trypan blue and counted in triplicate wells. No significant change in the number of single cells reflects impaired formation of desmosomes. Scale bars, 1 mm. Error bars represent s.d., t -test P value *<0.05; two-way analysis of variance ***<0.001). Full size image None of the downregulated mRNAs ( Supplementary Fig. 3B ) has been reported as direct transcriptional target of Nrf2. Since miR-29a and miR-29b were the only miRs upregulated in the skin of K5Cre-CMVcaNrf2 mice, we hypothesized that a miR-29-mediated downregulation of desmosomal proteins affects the formation of desmosomes in keratinocytes. We tested this hypothesis by performing in vitro cell aggregation assays in immortalized, but non-tumorigenic human epidermal keratinocytes (HaCaT cells) cultured at low calcium concentration for several passages to limit differentiation and concomitant formation of hyper-adhesive desmosomes [34] . Before the induction of desmosome formation and cell aggregation by increasing concentrations of calcium, cells were transfected with miR-29a or miR-29b mimics and incubated for 72 h. After detachment and filtering, the resulting single-cell suspensions were further cultured at different concentrations of extracellular calcium. On increase in the calcium concentration, HaCaT cells form hyper-adhesive desmosomes and rapidly clump together [34] . Transfection and 3-day incubation of the cells with miR-29a or miR-29b mimics impaired the formation of hyper-adhesive desmosomes as reflected by reduced clumping and enhanced release of single cells into the medium on shaking ( Fig. 4d ). This result demonstrates that increased levels of miR-29 inhibit formation of hyper-adhesive desmosomes in vitro and thus provides an explanation for the structural alterations of the desmosomes found in K5Cre-caNrf2 mice in vivo . Nrf2 regulates Dsc2 via miR-29s We next analysed RNA microarray data from skin of K5Cre and K5Cre-CMVcaNrf2 mice for RNAs, which encode desmosomal proteins and which are downregulated in the presence of caNrf2. The most strongly downregulated mRNA of this class encodes the desmosomal cadherin Dsc2 ( Supplementary Fig. 3B ), and miR-29s have their ‘seed’ sequence matching to the 3′UTR of both human and mouse Dsc2 mRNAs ( Supplementary Fig. 4A ). Transfection of HaCaT cells and primary human keratinocytes with miR-29a or miR-29b mimics significantly decreased the levels of DSC2 mRNA and protein ( Fig. 5a,b ). The effect of miR mimics on the expression of DSC2 was independent of their concentration in the range of 1–50 nM ( Supplementary Fig. 4B ), suggesting that the functional pool of transfected mimics is limited by their binding to Argonaute proteins [35] . Therefore, the amount of RISC-associated miR-29s in the transfected cells is comparable to the levels of abundant endogenous miRNAs [35] . Transfection with antagomiRs that specifically bind and decrease levels of miR-29a, miR-29b and miR-29c resulted in a significant increase in DSC2 mRNA ( Fig. 5c ) and protein levels ( Fig. 5d ), demonstrating that endogenous miR-29 also regulates DSC2. We next used miR-29 antagomiRs to determine if reduction of the levels of these miRs after activation of NRF2 in human keratinocytes rescues expression of DSC2. Treatment of HaCaT cells with compound 1a significantly decreased the levels of DSC2 mRNA ( Fig. 5e and Supplementary Fig. 4C ), which was prevented by transfection with miR-29 antagomiRs ( Fig. 5e and Supplementary Fig. 4D ). Similarly, treatment with miR-29 antagomiRs rescued the reduced expression of Dsc2 observed in two independent pools of primary mouse keratinocytes isolated from K5Cre and K5Cre-CMVcaNrf2 mice ( Supplementary Fig. 4E ). 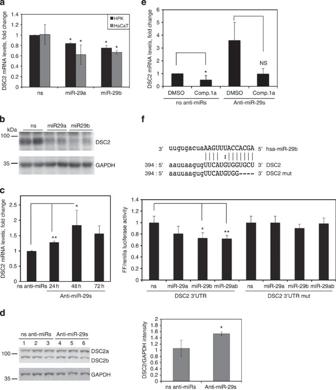Figure 5: miR-29s regulate the expression of DSC2 in human keratinocytes. (a) Levels ofDSC2mRNA in human primary keratinocytes (HPK) and HaCaT cells transfected with miR-29 mimics or non-specific (scrambled) oligonucleotides (ns). mRNA levels were measured by qRT-PCR and calculated as fold change over control (N=3). (b) Protein levels of DSC2 in corresponding HaCaT cells transfected with miR-29s or scrambled oligonucleotides were analysed by Western blot. (c,d) Levels of DSC2 mRNA (c) and protein (d) on transfection of HaCaT keratinocytes with antagomiRs targeting miR-29a, miR-29b and miR-29c (combined transfection) or scrambled (non-specific; ns) sequences. Cells were collected at indicated time points post transfection; ns set as 1 for each time point (N=3). (e)DSC2mRNA was quantified in HaCaT cells transfected with antigomiR-29s and non-specific antagomiRs before treatment with compound1a(25 μM) to activate NRF2 (N=3). (f) Human embryonic kidney cells were transfected with plasmids harbouring the full-length wild-typeDSC23′UTR or the 3′UTR with a mutation in the miR-29 binding site downstream of the luciferase coding region together with miR-29 mimics or non-specific controls. Lysates were analysed for luciferase activity (N=3). Error bars represent s.d.,Pvalue *<0.05; **<0.01. RT–PCR, reverse transcriptase-PCR. Figure 5: miR-29s regulate the expression of DSC2 in human keratinocytes. ( a ) Levels of DSC2 mRNA in human primary keratinocytes (HPK) and HaCaT cells transfected with miR-29 mimics or non-specific (scrambled) oligonucleotides (ns). mRNA levels were measured by qRT-PCR and calculated as fold change over control ( N =3). ( b ) Protein levels of DSC2 in corresponding HaCaT cells transfected with miR-29s or scrambled oligonucleotides were analysed by Western blot. ( c , d ) Levels of DSC2 mRNA ( c ) and protein ( d ) on transfection of HaCaT keratinocytes with antagomiRs targeting miR-29a, miR-29b and miR-29c (combined transfection) or scrambled (non-specific; ns) sequences. Cells were collected at indicated time points post transfection; ns set as 1 for each time point ( N =3). ( e ) DSC2 mRNA was quantified in HaCaT cells transfected with antigomiR-29s and non-specific antagomiRs before treatment with compound 1a (25 μM) to activate NRF2 ( N =3). ( f ) Human embryonic kidney cells were transfected with plasmids harbouring the full-length wild-type DSC2 3′UTR or the 3′UTR with a mutation in the miR-29 binding site downstream of the luciferase coding region together with miR-29 mimics or non-specific controls. Lysates were analysed for luciferase activity ( N =3). Error bars represent s.d., P value *<0.05; **<0.01. RT–PCR, reverse transcriptase-PCR. Full size image To validate the predicted binding sites of miR-29s in the 3′UTR of the DSC2 mRNA, we cloned the full-length 3′UTR region of the DSC2 mRNA into a luciferase reporter vector. Human embryonic kidney cells transfected with the 3′UTR reporter construct showed a significantly lower luciferase activity on co-transfection of miR-29a or miR-29b mimics compared with cells co-transfected with ns mimics ( Fig. 5f ). This reduction was not observed when cells were transfected with a luciferase construct containing the DSC2 3′UTR with a mutated miR-29 binding site ( Fig. 5f ). Thus, DSC2 is indeed a direct target of miR-29s. Taken together, these data demonstrate that Nrf2 regulates Dsc2 via miR-29 in mouse and human keratinocytes. Dsc2 controls formation of hyper-adhesive desmosomes The Nrf2-dependent downregulation of Dsc2 in the epidermis of K5CreCMV-caNrf2 mice ( Supplementary Fig. 3B ) was confirmed by quantitative reverse transcriptase-PCR ( Fig. 6a ). Importantly, the stronger downregulation at P32 (80%) compared with P2.5 (60%) correlates with the stronger expression of the caNrf2 transgene [9] . Suppression of Dsc2 expression by activated Nrf2 is a cell autonomous effect, since it was also observed in cultured primary keratinocytes from K5Cre-CMVcaNrf2 mice ( Fig. 6b ). The decrease in mRNA levels of Dsc2 translated into a dramatic reduction of Dsc2 protein levels in the epidermis of K5Cre-CMVcaNrf2 mice ( Fig. 6c and Supplementary Fig. 5A ). Importantly, Dsc2 co-localized with desmoplakin, another desmosomal component ( Fig. 6c ) in the epidermis K5Cre mice, demonstrating that Dsc2 preferentially localizes to desmosomes. 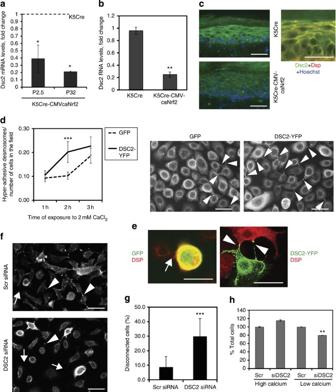Figure 6: Nrf2 regulates the expression of DSC2 in the epidermis and controls formation of hyper-adhesive desmosomes. (a) Levels of Dsc2 mRNA in total skin from K5Cre-CMVcaNrf2 mice and control littermates (N=3) at P2.5 and P32. Levels in control mice were set as 1 for each time point (dashed line). (b) Levels of Dsc2 mRNA in primary keratinocytes from K5Cre-CMVcaNrf2 mice and control littermates (N=4) isolated from epidermis at P4.5. (c) Tail skin of K5Cre and K5Cre-CMVcaNrf2 mice was stained with antibodies against Dsc2 (green; left and right panel) and desmoplakin (Dsp, red, left panel). Yellow colour indicates co-localization of Dsc2 and Dsp in desmosomes at the cell–cell border in K5Cre epidermis. Scale bars, 20 μm. (d) HPKs were transfected with DSC2-YFP or GFP (control) expression vectors and exposed to 2 mM CaCl2for 1–3 h to induce the formation of desmosomes. After removal of CaCl2, the remaining hyper-adhesive, calcium-insensitive desmosomes were stained with a desmoplakin (DSP) antibody. The percentage of keratinocytes connected by calcium-insensitive, hyper-adhesive desmosomes among all keratinocytes was determined. Ten fields per dish with at least 100 cells per field were counted in three independent dishes for every time point. Representative images of keratinocytes 2 h after exposure to high CaCl2concentrations stained with a DSP antibody. DSP in hyper-adhesive desmosomes is indicated with arrowheads. (e) DSC2-YFP (green) co-localizes with DSP (red) at the site of desmosome formation (arrowheads). Note that transfection with a GFP expression vector does not affect formation/function of desmosomes and that GFP does not co-localize with DSP at the cell membrane (arrow). (f) Formation or hyper-adhesive desmosomes by HaCaT cells under high calcium concentrations following transfection with scrambled (Scr) or DSC2 siRNA. Desmoplakin staining indicates hyper-adhesive desmosomes (arrowheads). Arrows point to single cells disconnected from neighbouring cells as a result of loss of hyper-adhesive desmosomes. (g) Quantification of disconnected cells following transfection with Scr or DSC2 siRNA and after treatment with ethylene glycol tetraacetic acid. At least 2,000 cells were counted in three independent dishes. (h) Total number of cells transfected with Scr or DSC2 siRNA and incubated in high or low calcium medium. Error bars represent s.d.,t-testPvalue *<0.05; **<0.01, ***<0.001. Figure 6: Nrf2 regulates the expression of DSC2 in the epidermis and controls formation of hyper-adhesive desmosomes. ( a ) Levels of Dsc2 mRNA in total skin from K5Cre-CMVcaNrf2 mice and control littermates ( N =3) at P2.5 and P32. Levels in control mice were set as 1 for each time point (dashed line). ( b ) Levels of Dsc2 mRNA in primary keratinocytes from K5Cre-CMVcaNrf2 mice and control littermates ( N =4) isolated from epidermis at P4.5. ( c ) Tail skin of K5Cre and K5Cre-CMVcaNrf2 mice was stained with antibodies against Dsc2 (green; left and right panel) and desmoplakin (Dsp, red, left panel). Yellow colour indicates co-localization of Dsc2 and Dsp in desmosomes at the cell–cell border in K5Cre epidermis. Scale bars, 20 μm. ( d ) HPKs were transfected with DSC2-YFP or GFP (control) expression vectors and exposed to 2 mM CaCl 2 for 1–3 h to induce the formation of desmosomes. After removal of CaCl 2 , the remaining hyper-adhesive, calcium-insensitive desmosomes were stained with a desmoplakin (DSP) antibody. The percentage of keratinocytes connected by calcium-insensitive, hyper-adhesive desmosomes among all keratinocytes was determined. Ten fields per dish with at least 100 cells per field were counted in three independent dishes for every time point. Representative images of keratinocytes 2 h after exposure to high CaCl 2 concentrations stained with a DSP antibody. DSP in hyper-adhesive desmosomes is indicated with arrowheads. ( e ) DSC2-YFP (green) co-localizes with DSP (red) at the site of desmosome formation (arrowheads). Note that transfection with a GFP expression vector does not affect formation/function of desmosomes and that GFP does not co-localize with DSP at the cell membrane (arrow). ( f ) Formation or hyper-adhesive desmosomes by HaCaT cells under high calcium concentrations following transfection with scrambled (Scr) or DSC2 siRNA. Desmoplakin staining indicates hyper-adhesive desmosomes (arrowheads). Arrows point to single cells disconnected from neighbouring cells as a result of loss of hyper-adhesive desmosomes. ( g ) Quantification of disconnected cells following transfection with Scr or DSC2 siRNA and after treatment with ethylene glycol tetraacetic acid. At least 2,000 cells were counted in three independent dishes. ( h ) Total number of cells transfected with Scr or DSC2 siRNA and incubated in high or low calcium medium. Error bars represent s.d., t -test P value *<0.05; **<0.01, ***<0.001. Full size image The reduction in Dsc2 expression in the epidermis of K5Cre-CMVcaNrf2 mice provides a likely explanation for the loss of the midline in most of the epidermal desmosomes of these mice ( Fig. 4c ), since midline formation correlates with hyper-adhesiveness [36] and since protein levels of DSC2 specifically increased at the time of the formation of hyper-adhesive desmosomes [34] . To further test this possibility, we transfected human primary keratinocytes with a DSC2-yellow fluorescent protein (YFP) expression vector or a green fluorescent protein (GFP) control vector. Primary keratinocytes do not form hyper-adhesive desmosomes within the first days of culturing in low calcium medium, thus providing an optimal system to study an inducible hyper-adhesiveness [37] . The number of hyper-adhesive desmosomes strongly increased in cells transfected with the DSC2-YFP plasmid compared with cells transfected with the GFP control vector within the first 2 h after exposure to high calcium concentrations ( Fig. 6d ). With the onset of stratification after 3 h of calcium treatment [37] , the number of hyper-adhesive desmosomes increased in all samples ( Fig. 6d ). DSC2-YFP was detected at the sites of hyper-adhesive desmosomes and co-localized with desmoplakin ( Fig. 6e ). Despite increased levels of DSC2-YFP and the higher number of hyper-adhesive desmosomes in transfected cells, the levels of desmoplakin did not change ( Supplementary Fig. 5B ), suggesting that upregulation of DSC2 protein alone is insufficient to change the total number of desmosomes. However, it affects the function of desmosomes through increasing their hyper-adhesiveness. To determine if a decrease of DSC2 levels has the opposite effect, we knocked down DSC2 and tested desmosome formation at high calcium concentrations, a physiologic condition under which desmosomes become hyper-adhesive and maintain the integrity of the epidermis [33] . HaCaT cells were used for this purpose, since they express high levels of DSC2, form hyper-adhesive desmosomes and provide a useful system to test the effect of DSC2 downregulation on hyper-adhesiveness. Cells were transfected with siRNA against DSC2 or control siRNA (for knock-down verification see Supplementary Fig. 5C ) and grown in high calcium medium until they formed hyper-adhesive, calcium-insensitive desmosomes [34] . The number of hyper-adhesive desmosomes was estimated on removal of calcium from the medium and staining with a desmoplakin antibody, which shows single bright dots only between cells connected by hyper-adhesive desmosomes ( Fig. 6f,g ) [34] . The number of disconnected cells was significantly higher after transfection with DSC2 siRNA ( Fig. 6f,g ), indicating that fewer hyper-adhesive desmosomes had formed after DSC2 knockdown. Although siRNA transfection did not affect cell proliferation ( Fig. 6h , high calcium conditions), a strong DSC2 knockdown resulted in a partial loss of cells from the culture dish under low calcium conditions ( Fig. 6h ). Thus, we observed a reduced number of connected cells on DSC2 knockdown ( Fig. 6f ), most likely due to a weaker initial cell–cell attachment on the dish as a result of desmosomal alterations. This finding demonstrates that downregulation of DSC2 reduces cell–cell adhesiveness by affecting the hyper-adhesive state of desmosomes and that the suppression of Dsc2 expression by Nrf2 is indeed functionally important by affecting hyper-adhesiveness of epidermal desmosomes. We present here a novel role of Nrf2 in the control of desmosome function. A basal activity of Nrf2 appears to support formation of hyper-adhesive desmosomes between keratinocytes, whereas further activation of Nrf2 resulted in the formation of enlarged desmosomes in vivo . Importantly, most desmosomes lacked the midline that is characteristic for hyper-adhesive desmosomes [33] , [38] . A combination of expression data, bioinformatics and functional assays strongly suggest that the midline abnormalities that we observed in vivo result from suppression of Dsc2 expression on activation of Nrf2. Dsc2 is a major component of desmosomes, and homozygous frameshift mutations in the DSC2 gene cause the syndrome of arrhythmogenic right ventricular cardiomyopathy, mild palmoplantar keratoderma and woolly hair [39] . Despite its clinical significance, the mechanisms of DSC2 regulation and its specific role in desmosome formation and/or maturation are largely unknown. Earlier in situ hybridization analysis of human skin demonstrated DSC2 expression in most layers of the epidermis, and the intensity of the DSC2 signal in basal and suprabasal cells was higher compared with other types of DSC. This finding suggested an involvement of DSC2 in the formation of hyper-adhesive desmosomes during keratinocyte differentiation [40] . The in vivo expression data in the mouse and the functional data presented here support this hypothesis and strongly argue for a non-redundant role of Dsc2 in desmosome maturation during stratification. A reduction in hyper-adhesion as a consequence of reduced Dsc2 expression is expected to affect epidermal homeostasis, because hyper-adhesive desmosomes are more strongly adhesive than calcium-dependent desmosomes [34] . Indeed, K5Cre-CMVcaNrf2 mice have significantly reduced levels of Dsc2 protein in the epidermis. These mice develop impaired barrier function as a result of abnormalities in the cornified envelope [9] , and the desmosomal abnormalities are likely to contribute to this impairment. Reduction of Dsc2 levels may also affect cell mobility, since loss of hyper-adhesion is associated with wound re-epithelialization and since downregulation of DSC2 promoted invasiveness of oral squamous cell carcinoma cells [36] , [41] , [42] . Our results further demonstrate that the Nrf2-mediated suppression of Dsc2 expression is dependent on miR-29a and -b, which are upregulated in response to genetic or pharmacological activation of Nrf2 in keratinocytes and which directly target the Dsc2 mRNA. This novel Nrf2-miR-29-Dsc2 axis is functionally important, since siRNA-mediated downregulation of DSC2 or overexpression of miR-29a/b impaired the formation of functional desmosomes in cultured keratinocytes, whereas overexpression of DSC2 had the opposite effect. Therefore, activation of Nrf2 and consequently, a miR-29-dependent reduction of Dsc2 levels, are likely to interfere with the formation of hyper-adhesive desmosomes in the skin of K5Cre-CMVcaNrf2 mice. Our data provide first evidence for a regulation of DSC2 by miRNAs. This finding is consistent with the important role of miRNAs in the control of cell–cell and cell–matrix adhesion [43] . The length of the Dsc2/DSC2 3′UTR allows for binding of additional miRNAs; therefore, the strong downregulation of Dsc2 expression in the skin of K5Cre-CMVcaNrf2 mice as compared with a relatively mild downregulation of DSC2 by miR-29s in culture may be explained by the synergistic binding of several miRNAs to the 3′UTR of Dsc2 in vivo . miR-29s are important regulators of cell–matrix adhesion [44] , [45] , and our data extend the role of these miRNAs to the control of cell–cell adhesion. By combining in silico and microarray analyses, we identified at least 4,707 mRNAs that are expressed in the skin and are potentially regulated by miR-29 through binding to their 3′UTRs. Only 71 of them are validated miR-29 targets, whereas the others await further investigation. These findings suggest various additional functions of miR-29s in skin biology, which remain to be identified. The proteins encoded by these mRNAs control various pathways, and their potential roles in cancer are particularly intriguing. This is important with regard to the enhanced activity of NRF2 in various types of human cancer [6] , [7] . Our ChIP experiments revealed that the Mir29ab1 and Mir29b2c genes are direct targets of endogenous Nrf2 as well as of transgene-derived caNrf2 and dnNrf2 in vitro and in vivo . The identification of these Nrf2-regulated miRs is in line with data from a recent ChIP-Seq experiment, which identified >15,000 Nrf2-bound sites in hepatoma cells [46] . The majority of them are located within mRNA-coding genes or intergenic regions and constitute >92% of all Nrf2-bound sites genome wide [46] . Since genes coding for miRNAs are located either within open reading frames of mRNA genes or in intergenic ‘desert’ regions, these data strongly suggest a function of Nrf2 as a regulator of genes coding for miRNAs. In this study, we demonstrate that binding of Nrf2 to the AREs in the 5′-region of miRNA genes is functionally important, since it resulted in upregulation of miR-29 expression. We also show that only binding of Nrf2 to the Mir29ab1 cluster of the mouse and human genome resulted in transcriptional activation. Analysis of histone modifications around the Nrf2-bound Mir29ab1 ARE confirmed that the site serves as an active enhancer. Importantly, the activation of this enhancer is dependent on the transactivation domain of Nrf2, since binding of dnNrf2 reduced the H3K4me2 modification and failed to activate the Mir29ab1 gene. In contrast, binding of Nrf2 to the Mir29b2c ARE is obviously not sufficient to activate transcription of this gene cluster in keratinocytes, since it was silenced by DNA methylation of the promoter region. Prevention of NRF2-mediated activation by DNA methylation in the promoter region was also shown for the p66 Shc gene in human lung cancer cells [47] . Another NRF2 ChIP-Seq study using human lymphoblastoid cells confirmed the genome-wide distribution of NRF2 binding in the vicinity of miRNA genes and found a peak of NRF2 binding in the upstream region of the human MIR29AB1 cluster [14] . Surprisingly, however, treatment of these lymphoblastoid cells with the NRF2-activating compound sulforaphane resulted in a downregulation of mature miR-29b (ref. 14 ). The discrepancy to our results obtained in keratinocytes may result from NRF2-independent effects of sulforaphane on expression/maturation of miR-29 (ref. 48 ) or from cell-type specific differences in the regulation of mature miRNAs. Consistent with this hypothesis, we found different effects of Nrf2 on the levels of mature miR-29s in keratinocytes versus several other cell types. Furthermore, sulforaphane caused only a minor upregulation of miR-29a and miR-29b in keratinocytes compared with the less toxic compound 1a . The identification of additional Nrf2-regulated miRNAs may lead to the discovery of Nrf2-mediated miRNA functions in different tissues and organs. Indeed, recent data showed that miRNAs that are downregulated in tumour cells with hyperactive NRF2 affect the metabolism of these cells [49] and that Nrf2-mediated upregulation of miR-125b suppresses expression of the aryl hydrocarbon receptor in the kidney [15] . Taken together, we unravelled a novel role of Nrf2 in the control of miRNA expression in keratinocytes and we show that an Nrf2-miR-29-Dsc2 axis controls desmosome function in the epidermis ( Fig. 7 ). These findings provide new insight into the mechanisms of Nrf2 action and help to explain how Nrf2 activation suppresses the expression of target genes. Our findings also revealed a novel interplay between DNA methylation and the Nrf2-mediated regulation of non-coding RNAs ( Fig. 7 ). Finally, we identified miRNAs as novel regulators of desmosomes. This finding is obviously important for the maintenance of epidermal barrier function and thus for cutaneous homeostasis. In the future, it will be interesting to determine if alterations in this new regulatory axis are associated with different human skin diseases. 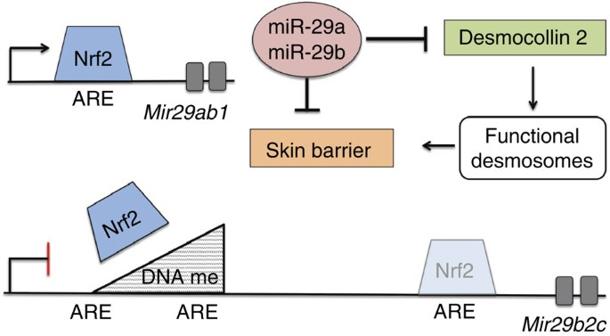Figure 7: Regulation and function of the Nrf2-miR-29-Dsc2 axis in the skin. Nrf2 directly induces expression of miR-29a and miR-29b in keratinocytes. This results in the suppression of Dsc2 expression and impairments in the formation of hyperactive desmosomes, which affects the skin barrier. In contrast, DNA methylation of the promoter of the lncRNA excludes functional binding of Nrf2 and likely prevents Nrf2-mediated activation of themiR29b2ccluster. Figure 7: Regulation and function of the Nrf2-miR-29-Dsc2 axis in the skin. Nrf2 directly induces expression of miR-29a and miR-29b in keratinocytes. This results in the suppression of Dsc2 expression and impairments in the formation of hyperactive desmosomes, which affects the skin barrier. In contrast, DNA methylation of the promoter of the lncRNA excludes functional binding of Nrf2 and likely prevents Nrf2-mediated activation of the miR29b2c cluster. Full size image Mouse maintenance and animal experimentation Transgenic mice expressing a caNrf2 mutant in keratinocytes [9] were housed under optimal hygiene conditions and maintained according to Swiss animal protection guidelines. All procedures with mice were approved by the local veterinary authorities of Zurich or Lausanne, Switzerland. Cell culture and transfection HaCaT cells and primary human keratinocytes were transfected with miR-29 MirVana mimics (Life Technologies, Carlsbad, CA) using Interferin transfection reagent (PolyPlus Transfection, Illkirch, France) according to the manufacturer’s instructions. Primary keratinocytes were isolated from newborn and adult mice using an overnight incubation with cold solution of dispase in PBS [50] . Primary human foreskin keratinocytes were obtained from healthy donors (obtained anonymously from the Department of Dermatology, University Hospital Zurich, in the context of the Biobank project, approved by the local and cantonal Research Ethics Committees) and cultured in keratinocyte-defined medium (K-SFM) with supplements (Life Technologies) [50] . A DSC2-YFP plasmid (kindly provided by Dr Rudolf Leube, RWTH Aachen) was used for transfection of primary human keratinocytes using Lipofectamine 2,000 (Life Technologies). Transfection with siRNA against DSC2 (Sigma, Munich, Germany) was performed according to the manufacturer’s protocol using RNA iMAX (Life Technologies). ChIP analysis Epidermis was separated from dermis by treatment of mouse skin with dispase. Chromatin lysate was prepared by homogenization of the epidermis in a series of buffers, adopted from Farnham lab protocols, and modified to efficiently disrupt the epidermis (original protocol is available at http://farnham.genomecenter.ucdavis.edu/protocol.html ). Chromatin was precleared with ns IgG (4 μg) and incubated overnight with 4 μg of antibodies against Nrf2 ref. 28 or Santa Cruz, Santa Cruz, CA), histone H3 (Abcam, Cambridge, UK), histone H3K4me1/2/3, (Active Motif Inc., Carlsbad, CA), histone H3K27Ac (Abcam) or 5 μg of normal rabbit IgG (Millipore, Billerica, MA). The percentage of the input that was bound was calculated by the dCt method and averaged over at least three experiments. Cell aggregation assays Cell aggregation assays, which allow overall estimation of desmosome formation before they become calcium-insensitive, were performed essentially as described previously [51] . Briefly, HaCaT cells transfected with miR-29a/b or ns mimics and incubated for 72 h. Cells were washed 3 × with ethylene glycol tetraacetic acid-containing medium to remove calcium, trypsinized, pressed through a 70-micron strainer to create a single-cell suspension and incubated in fresh medium with 0.05 and 0.25 mM CaCl 2 for 1 h. On formation of desmosomes, cells form clumps and sheets, thereby decreasing the number of single cells in suspension. Single cells were then stained with Trypan blue and counted in triplicate wells. No significant change in the number of single cells reflects impaired formation of functional desmosomes. Immunofluorescence staining of mouse skin Frozen sections of mouse tail skin (7 μm) were incubated with antibodies against mouse Dsc2 (R&D Systems, Minneapolis, MN) or desmoplakin [52] together with Hoechst to counterstain nuclei. Antibody-bound cells were detected with FITC-coupled sheep anti-rabbit antibody (Millipore) and Cy3-coupled goat anti-mouse secondary antibody (Jackson ImmunoResearch, West Grove, PA). Analysis of hyper-adhesive desmosomes Human keratinocytes transfected with DSC2-YFP or GFP expression vectors, and HaCaT cells transfected with siRNA against DSC2 or scrambled control were cultured in 2 mM CaCl 2 for 1–3 h (primary keratinocytes) or overnight (HaCaT cells). After reaching confluency and on exposure to high concentrations of calcium (2 mM), keratinocytes form hyper-adhesive desmosomes, which become calcium insensitive and resist the disruption by incubation in ethylene glycol tetraacetic acid [34] . These hyper-adhesive calcium-insensitive desmosomes were visualized by immunofluorescence staining with a desmoplakin antibody [52] . In low calcium medium, the concentration of Ca 2+ was <0.1 mM. DNA methylation analysis Genomic DNA was isolated from the epidermis of wild-type mice (8 weeks of age), HaCaT cells or primary human keratinocytes using the QiAmp DNA blood Mini kit (Qiagen, Hilden, Germany). Methylated DNA was precipitated using a mouse monoclonal antibody against 5-methylcytosine [53] and quantified using primers for the CpG regions of the A330023F24Rik/Mir29b2c and C1ORF132/MIR29B2C genes. Primers for the imprinted gene Dpep3 and UBE2B served as positive controls, whereas the Tbx15 and TSH2B genes void of DNA methylation served as a negative control [53] . For pyrosequencing analysis, 1 μg of the same sonicated DNA sample used for MeDIP was bisulfite modified using the EpiTect bisulfite kit (Qiagen). Bisulfite-modified DNA (2 μl) was used for the PCR analysis using biotin labelled pyrosequencing primers designed with the Pyro CpG software (Qiagen). PCR products were sequenced using the PyroMark Q96 instrument (Qiagen). For bisulfite conversion and sequencing of the human C1ORF132 CpG region (exon2-intron2), the 238 bp PCR product containing 25 CpGs was cloned into the pDRIve vector (Qiagen) and 10 colonies were sequenced. The in vitro methylated DNA was cloned and sequenced as a positive control and the unmethylated DNA was used as a negative control (Qiagen). The data was analysed using BISMA bioinformatics package ( http://www.biomedcentral.com/1471-2105/11/230 ). To study the relevance of methylation for gene expression, HaCaT cells and primary human keratinocytes were treated with 5-aza-2′deoxyuridine or solvent DMSO for 5 days with daily change of medium containing 0.5 μM (HaCaT cells) or 1 μM (primary keratinocytes) of 5-aza-2′deoxyuridine. Cloning and reporter assay and in vitro DNA methylation assay DSC2 3′UTR and DSC2 3′UTRmut were cloned into the pmirGLO dual reporter vector (Promega, Madison, WI) and used for transfection of human embryonic kidney cells following treatment with miR-29 or ns mimics for 24 h. The putative Nrf2 enhancer element of Mir29b2c including the ARE was inserted into the pGL4 vector with minimal promoter (minP) (Promega). An 8xARE-containing plasmid served as a positive control for the detection of Nrf2-mediated gene expression [29] . The CpG-free, promoter/enhancer free pCpGL vector [54] was used to clone the promoter of A330023F24Rik . In vitro DNA methylation assays were done using CpG-free pCpGL vector as described in ref. 54 with the CMV-pCpGL vector as a positive control. Plasmids were methylated using SssI methylase (New England Biolabs, Frankfurt am Main, Germany) according to the manufacturer’s instruction in the presence of S-Adenosylmethionine (New England Biolabs) for 4 h at 37 °C. The completeness of methylation was controlled by digesting both methylated and unmethylated DNA using methylation sensitive restriction enzymes HhaI and HpaII and methylation insensitive MspI. Purified plasmids were co-transfected together with a control plasmid containing the Renilla gene to HEK293 cells, and luciferase activity was measured using Dual-Glo luciferase assay kit (Promega) and a 96-well plate luminometer (Tecan, Maennedorf, Switzerland). Electron microscopy Mice were lethally anaesthetized with pentobarbital (700 mg kg −1 ) and perfused with 4% paraformaldehyde in PBS. Skin samples were fixed overnight in a 4% paraformaldehyde at 4 °C, rinsed and stored in PBS. After washing in 0.1 M cacodylate buffer pH 7.2 at 4 °C, the specimens were treated with 2% OsO 4 for 2 h. Afterwards they were washed, stained in 1% uranyl acetate, dehydrated through a series of graded ethanols and embedded in araldite resin. Ultra-thin sections (30–60 nm) were processed with a diamond knife and placed on copper grids. Transmission electron microscopy was performed using a 902A electron microscope (Zeiss, Oberkochen, Germany). qPCR and western blot analysis cDNA was synthesized from 2 μg total RNA using the iScript kit (Bio-Rad Laboratories, Hercules, CA). TaqMan qPCR for analysis of miRNAs was performed using specific primers and probes from Life Technologies. Antibodies against desmoplakin [55] and Dsc2 (Progen, Heidelberg, Germany) were used for western blot analysis at final dilution 1:500. Complete scans at the most important western blots are shown in Supplementary Figure 6 . Primers pa qRT-PCR are listed in Supplementary Table 1 . Bioinformatics analysis Potential binding sites for Nrf2 were searched among the gene promoter regions using the Match tool [56] . Match uses a library of mononucleotide weight matrices from TRANSFAC Professional (release 11.2.). The weight matrix search was performed using a cut-off that minimizes the sum of both false positive and negative error rates. Statistical analysis Results are expressed as mean ±s.d. Statistical analysis was performed using t -test, * P ≤0.05, ** P ≤0.01, *** P ≤0.001. Differences between groups that were not labelled with asterisks were non-significant. Two-way analysis of variance was used to estimate the difference of the desmosomal thickness. How to cite this article: Kurinna, S. et al . A novel Nrf2-miR-29-desmocollin-2 axis regulates desmosome function in keratinocytes. Nat. Commun. 5:5099 doi: 10.1038/ncomms6099 (2014).